Correlating interfacial octahedral rotations with magnetism in (LaMnO3+δ)N/(SrTiO3)Nsuperlattices Lattice distortion due to oxygen octahedral rotations have a significant role in mediating the magnetism in oxides, and recently attracts a lot of interests in the study of complex oxides interface. However, the direct experimental evidence for the interrelation between octahedral rotation and magnetism at interface is scarce. Here we demonstrate that interfacial octahedral rotation are closely linked to the strongly modified ferromagnetism in (LaMnO 3+ δ ) N /(SrTiO 3 ) N superlattices. The maximized ferromagnetic moment in the N =6 superlattice is accompanied by a metastable structure (space group Imcm ) featuring minimal octahedral rotations ( a − a − c − , α ~4.2°, γ ~0.5°). Quenched ferromagnetism for N <4 superlattices is correlated to a substantially enhanced c axis octahedral rotation ( a − a − c − , α ~3.8°, γ ~8 ° for N= 2). Monte–Carlo simulation based on double-exchange model qualitatively reproduces the experimental observation, confirming the correlation between octahedral rotation and magnetism. Our study demonstrates that engineering superlattices with controllable interfacial structures can be a feasible new route in realizing functional magnetic materials. Oxides interface offers a remarkably rich playground for creating new quantum states and functional properties utilizing different interfacial reconstruction mechanisms. Extensive studies have been focused on introducing novel physical properties at the interface [1] , [2] . Recently, oxygen octahedral rotation (OOR) manipulation in artificial superlattices was made possible through accurate OOR detection based on cutting-edge scanning transmission electron microscopy [3] , [4] and synchrotron X-ray diffraction (XRD) [5] , [6] . First-principles calculations have demonstrated that interface OOR can be altered or entirely different from the bulk phase by proximity effects, electronic instabilities or OOR-strain coupling [7] , [8] , [9] , [10] . Since the metal–oxygen bonds have an important role in determining the orbital order and exchange interactions, novel magnetic modulations are expected as a result of new interface OOR. Earlier experiments have found that novel magnetic properties such as high-temperature antiferromagnetic phase [11] and uniaxial magnetic anisotropy [12] , [13] in ultrathin oxide films could be explained by lattice symmetry changes associated with different OOR patterns. However, a comprehensive study to accurately determine the OOR and its role in the interface magnetic structure has not been attained and is therefore pressing. We conducted a combined experimental and theoretical study to find the correlation between the OOR and the magnetic properties in (LaMnO 3+ δ ) N /(SrTiO 3 ) N ( N =2, 3, 4, 6, 8, 16) superlattices. The maximized ferromagnetic (FM) moment is found in the N =6 superlattice accompanied by minimal octahedral rotations. Quenched FM for N <4 superlattices is correlated to a substantially enhanced c axis octahedral rotation. Monte–Carlo simulation qualitatively reproduces the experimental observation, and suggests that the OOR is strongly correlated to the double-exchange interaction. Details of the sample growth, the measurements and theoretical calculation are described in Methods section. At room temperature, bulk LaMnO 3+ δ exhibits either orthorhombic structure with a − a − c + type octahedral rotation (if Mn valence is close to 3+), or rhombohedra structure with a − a − a − rotation (if Mn valence is higher) [14] , [15] , [16] , [17] . SrTiO 3 in bulk exhibits a cubic structure above 105 K with no octahedral rotations. The details of the Glazer notation can be found in ref. 18 . The strong symmetry breaking at the interface makes the LaMnO 3+ δ /SrTiO 3 superlattice a prototypical system to investigate the impact of interface OOR misfit. 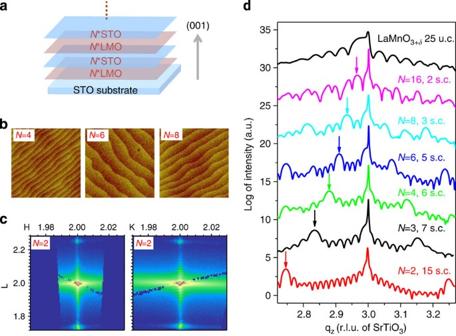Figure 1: Characterization of (LaMnO3+δ)N/(SrTiO3)Nsuperlattices grown on SrTiO3(001) substrate. (a) The stacking order of LaMnO3+δ(LMO) and SrTiO3(STO) in the superlattices; (b) 2 × 2 μm2atomic force microscopy images forN=4, 6, 8 superlattices; (c)HL(left) andKL(right) reciprocal space maps near (H,K,L)=(2,2,2) for theN=2 superlattice. The intensity is shown on a logarithmic scale. The slanted lines that cut through the SrTiO3Bragg peak are because of the insertion of attenuators for X-ray measurements near Bragg peaks. (d) Specular XRD data (H,K=0) for all the superlattices with different periodNand supercell (s.c.) numbers nearL=3, in reciprocal lattice units (r.l.u.) of SrTiO3. The spectra are vertically shifted for clarity. The peaks associated with the superlattice modulation are indicated by arrows. The data from a 25 unit cell (u.c.) LaMnO3+δfilm is also shown for reference. Interface structure and magnetic properties Figure 1a shows the schematic stacking order of (LaMnO 3+ δ ) N /(SrTiO 3 ) N superlattices grown on (001) SrTiO 3 substrates. The atomic force microscopy images in Fig. 1b reveal smooth terraces on superlattice surfaces with typical roughness of 1.5 Å. The sharp interfaces with roughness smaller than 2 Å are confirmed from the low-angle X-ray reflectivity ( Supplementary Fig. 1a ). All superlattices are coherently strained to SrTiO 3 substrates ( Fig. 1c and Supplementary Fig. 2 ). Figure 1d shows the specular rods ( H = K =0) for all superlattices and a reference LaMnO 3+ δ thin film. Pronounced thickness fringes with well-defined superlattice peaks (indicated by arrows) can be clearly observed and their positions agree well with the expected values based on the reflection high-energy electron diffraction (RHEED) oscillations, confirming the high-quality epitaxy and smoothness of the interface. Figure 1: Characterization of (LaMnO 3+ δ ) N /(SrTiO 3 ) N superlattices grown on SrTiO 3 (001) substrate. ( a ) The stacking order of LaMnO 3+ δ (LMO) and SrTiO 3 (STO) in the superlattices; ( b ) 2 × 2 μm 2 atomic force microscopy images for N =4, 6, 8 superlattices; ( c ) HL (left) and KL (right) reciprocal space maps near ( H , K , L )=(2,2,2) for the N =2 superlattice. The intensity is shown on a logarithmic scale. The slanted lines that cut through the SrTiO 3 Bragg peak are because of the insertion of attenuators for X-ray measurements near Bragg peaks. ( d ) Specular XRD data ( H , K =0) for all the superlattices with different period N and supercell (s.c.) numbers near L =3, in reciprocal lattice units (r.l.u.) of SrTiO 3 . The spectra are vertically shifted for clarity. The peaks associated with the superlattice modulation are indicated by arrows. The data from a 25 unit cell (u.c.) LaMnO 3 + δ film is also shown for reference. Full size image The magnetic properties are shown in Fig. 2a–c . Bulk stoichiometric LaMnO 3 exhibits A-type antiferromagnetic order with a spin moment of 4 μ B per Mn site. The thin films usually exhibit weak FM with the chemical composition of LaMnO 3+ δ due to cation vacancies or strain effect [19] , [20] , [21] , [22] , [23] . If interfacial magnetic reconstructions are absent, M s (saturation magnetization) of the superlattices should be same as that of the reference LaMnO 3+ δ thin film ( M s *), and T c (FM transition temperature) should slowly decrease with T c * (α J ex ν , mean-field estimate owing to less neighbouring MnO 2 planes at the interface; J ex is the exchange energy and ν is the number of nearest Mn atoms.). The N =16 superlattice follows the simple estimate of M s * and T c *, but the N <16 superlattices exhibit large deviations from the estimate. In particular, the N =6 superlattice exhibits a maximal M s of 2.97 μ B /Mn, whereas the N =2 superlattice exhibits distinctly quenched FM with T c =25 K and M s =1.14 μ B /Mn. In Fig. 2b , the N =2, 3, 4 superlattices exhibit small shoulders below 15 K possibly originating from weak Ti FM [24] . The non-monotonic relationship between M s and the period N indicates a complex interplay between the multiple degrees of freedom (lattice-charge-spin-orbital). 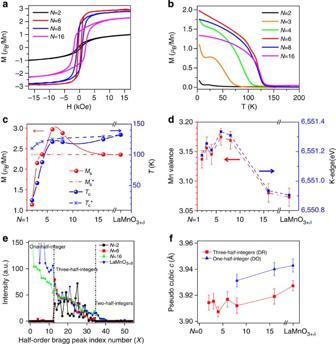Figure 2: Correlation between magnetic and structural properties of the (LaMnO3+δ)N/(SrTiO3)Nsuperlattices. (a) The hysteresis loops measured atT=4 K along the in-plane direction. (b) The magnetization as a function of temperature measured after field cooling along the in-plane direction. The cooling field was 1,000 Oe and the magnetization was measured during warming up in a field of 100 Oe. (c) The saturation magnetization (Ms) and the FM transition temperature (Tc) as a function of the superlattice periodN.Ms* andTc* are the mean-field estimates without the presence of interfacial reconstructions. (d) The Mn K-edge threshold energy measured from XAFS and the derived Mn valence (see Methods section). (e) Half-order Bragg peak intensity for four representative samples (N=2, 6, 16 and LaMnO3+δfilm). Each point in the data corresponds to one certain half-order Bragg peak with assigned indexX, whoseHKLvalues can be found inSupplementary Table 1. Half-order peaks with theirXindex ranging from [0,12], [13,34] and [35,55] correspond to peaks with one ofH,K,Lhalf-integer, peaks with all three-half-integers, and peaks with two-half-integers, respectively. (f) Pseudocubic lattice constant along thecaxis (cp) as a function of superlattice periodicityNdeduced from half-order Bragg peaks. The results for two types of half-order peaks, representing DR and DO phase, respectively, are generated by averaging all measured peaks. The error bars indicate statistical variance. Figure 2: Correlation between magnetic and structural properties of the (LaMnO 3+ δ ) N /(SrTiO 3 ) N superlattices. ( a ) The hysteresis loops measured at T =4 K along the in-plane direction. ( b ) The magnetization as a function of temperature measured after field cooling along the in-plane direction. The cooling field was 1,000 Oe and the magnetization was measured during warming up in a field of 100 Oe. ( c ) The saturation magnetization ( M s ) and the FM transition temperature ( T c ) as a function of the superlattice period N . M s * and T c * are the mean-field estimates without the presence of interfacial reconstructions. ( d ) The Mn K-edge threshold energy measured from XAFS and the derived Mn valence (see Methods section). ( e ) Half-order Bragg peak intensity for four representative samples ( N =2, 6, 16 and LaMnO 3+ δ film). Each point in the data corresponds to one certain half-order Bragg peak with assigned index X , whose HKL values can be found in Supplementary Table 1 . Half-order peaks with their X index ranging from [0,12], [13,34] and [35,55] correspond to peaks with one of H , K , L half-integer, peaks with all three-half-integers, and peaks with two-half-integers, respectively. ( f ) Pseudocubic lattice constant along the c axis ( c p ) as a function of superlattice periodicity N deduced from half-order Bragg peaks. The results for two types of half-order peaks, representing DR and DO phase, respectively, are generated by averaging all measured peaks. The error bars indicate statistical variance. Full size image Mn valence analysis We performed X-ray absorption fine structure (XAFS) measurements at the Mn K-edge to probe its valence change. The K-edge threshold energy continuously increases with increasing Mn valence [25] . Details of the XAFS analysis are given in the Methods section and Supplementary Fig. 3 . The derived Mn valences are shown in Fig. 2d . The Mn valence exhibits a sudden drop for N >8, but stays more or less constant for N <8. The increased Mn valence can be explained by electron leaking from LaMnO 3+ δ to SrTiO 3 that enhances the FM magnetization. Such charge transfer phenomena have been observed at previous LaMnO 3 /SrTiO 3 interfaces although the detailed mechanism differ in different samples [26] , [27] , [28] , [29] . However, the strongly suppressed FM for N <4 cannot be explained by the valence change alone, because Mn valences in these superlattices are fairly high (~+3.14), and, in particular, much higher than that of the N =16 superlattice or the LaMnO 3+ δ thin film. Therefore, interfacial reconstruction mechanisms other than just charge transfer have to be invoked. Analysis of octahedral rotation from XRD It has been demonstrated that OOR gives rise to a unique XRD intensity profile of half-order peaks, allowing for accurate determination of the rotation angles [5] , [6] . Experimentally, we systematically measured 55 half-order Bragg peaks and labelled each with an index number X (the correspondence between X and its associated ( H , K , L ) values can be found in Supplementary Table 1 ). The measured intensities of these peaks are summarized in Fig. 2e for four representative samples, that is, the N =2, 6, 16 superlattices and the LaMnO 3+ δ film. Since bulk LaMnO 3+ δ exhibits strong OOR and bulk SrTiO 3 assumes an ideal cubic structure with no rotations at room temperature (where the XRD measurements were conducted), it is reasonable to believe that the half-order Bragg peaks originate mostly from LaMnO 3+ δ layers and (possibly) interfacial SrTiO 3 . All the peaks are classified into three types: peaks with one-half-integer and two integer indices (for example, ( H , K , L )=(0.5,1,2)), peaks with two-half-integer and one integer indices (for example, ( H , K , L )=(0.5,1.5,2)) and peaks with three-half-integer indices (for example, ( H , K , L )=(0.5,1.5,2.5)). For the N =2 and 6 superlattices, the one-half-integer and two-half-integer peaks are essentially absent, and the three-half-integer peaks exhibit very large intensity variations (up to almost two order of magnitude). This can be naturally explained by OOR without any in-phase (+) rotations [5] , [30] , while neither cation displacements nor cooperative Jahn–Teller distortion could give rise to such an intensity pattern ( Supplementary Fig. 4 and Supplementary Note 1 ). Owing to the biaxial strain from substrates, these layers actually assume distorted rhombohedral (DR) structures with a − a − c − rotations [5] , [6] . For the N =16 superlattice and the LaMnO 3+ δ film, the Mn valence is close to +3, and correspondingly, a distorted orthorhombic (DO) phase emerges with in-phase rotation around one of the in-plane axis [15] , [16] , [17] , [31] , [32] , resulting in obvious two-half-integer peaks. The observed one-half-integer peaks cannot be produced by OOR, and are probably caused by La displacements [31] , which are well known to occur in bulk orthorhombic phases [14] . The pseudocubic lattice constant along the c axis ( c p ) of the DR and DO phases, determined from the half-order peaks ( Supplementary Fig. 5 ), is summarized in Fig. 2f . The c p values derived from the three-half-integer peaks show a relatively small variation with N (within the experimental uncertainty), and are always smaller than those obtained from one-half-integer peaks. This suggests that c p obtained from three-half-integer peaks mostly originates from the DR phase, which is smaller due to larger Mn valences ( Fig. 2d ). The larger c p from one-half-integer peaks are attributed explicitly to the DO phase with Mn valence close to +3. The coexistence of the DR phase (stronger FM and probably near the interface) and DO phase (weaker FM and probably deep inside the LaMnO 3+ δ layer) in N ≥8 superlattices naturally explains the decrease of the FM moment. Since the half-order Bragg peaks in the N ≤6 superlattices are expected to arise from the a − a − c − OOR, the rotation angles could be determined by numerically fitting the intensity pattern according to the model in refs 5 , 6 . In this model, the positions of 24 oxygen atoms in a 2 × 2 × 2 supercell were individually calculated based on the OOR, and their X-ray scattering amplitudes were added up coherently to yield the best fit to the experimental peak intensities ( Supplementary Note 1 ). Indeed, we are able to obtain excellent fits to the experimental data and the results are summarized in Fig. 3a . Our fitting shows that the rotation angle α (around in-plane pseudocubic axis) increases by 0.4° from N =2 up to N =6, whereas the rotation angle γ around pseudocubic c axis decreases sharply from ~8° for N =2 to almost zero for N =6 ( Fig. 3b ). From the rotation angles in Fig. 3a , we can determine the in-plane and out-of-plane bond angles and lengths as shown in Fig. 3c (ref. 6 ). As the FM exchange interactions in manganites depends sensitively on the bond angle [33] , the marked reduction in in-plane bond angles for N <4 superlattices would decrease the amplitude for electron hops, and thereby suppress the FM order. 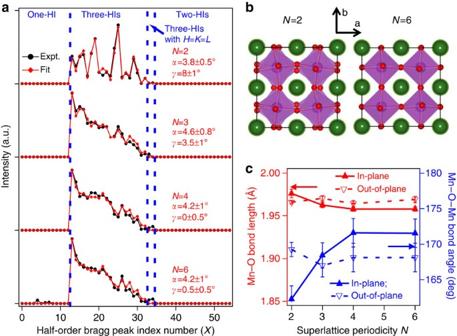Figure 3: Deducing the octahedral rotation forN=2–6 superlattice samples from the intensities of half-order Bragg peaks. (a) Experimental (Expt.) half-order Bragg peak intensities (black dots) compared with model fits (red diamonds). The Half-order Bragg peaks are again categorized by the index number (X), as defined inFig. 2e. Note that peaks atX=33, 34 correspond to three-half-integers (three-HIs) peaks withH=K=L. The rotation pattern isa−a−c−withαandγindicating the rotation angles aroundaandcaxis, respectively. The best fit values ofαandγare shown with error bars. The data and fits are shifted vertically for display clarity. (b) In-plane view, that is, top view, of the atomic structure model showing the fitted octahedral rotations for theN=2 andN=6 superlattices. Green, purple and red filled circles indicate La, Mn and O atoms, respectively. (c) In-plane (filled up triangles) and out-of-plane (hollow down triangles) Mn–O bond lengths (red) and Mn–O–Mn bond angles (blue) deduced from the octahedral rotation. The pseudocubic lattice constants are adapted fromFig. 2f. Figure 3: Deducing the octahedral rotation for N =2–6 superlattice samples from the intensities of half-order Bragg peaks. ( a ) Experimental (Expt.) half-order Bragg peak intensities (black dots) compared with model fits (red diamonds). The Half-order Bragg peaks are again categorized by the index number ( X ), as defined in Fig. 2e . Note that peaks at X =33, 34 correspond to three-half-integers (three-HIs) peaks with H = K = L . The rotation pattern is a − a − c − with α and γ indicating the rotation angles around a and c axis, respectively. The best fit values of α and γ are shown with error bars. The data and fits are shifted vertically for display clarity. ( b ) In-plane view, that is, top view, of the atomic structure model showing the fitted octahedral rotations for the N =2 and N =6 superlattices. Green, purple and red filled circles indicate La, Mn and O atoms, respectively. ( c ) In-plane (filled up triangles) and out-of-plane (hollow down triangles) Mn–O bond lengths (red) and Mn–O–Mn bond angles (blue) deduced from the octahedral rotation. The pseudocubic lattice constants are adapted from Fig. 2f . Full size image Double-exchange model simulation To establish a qualitative understanding between magnetism and OOR in our experiment, we performed a theoretical study based on the double-exchange model. We assume a clean system without charge non-stoichiometry and focus on the effect of OOR. The main physical effect of OOR to magnetism is the change of the Mn–O–Mn bond angles, as revealed in Fig. 3c , which tunes the exchange coefficients and bandwidth. To simulate this effect, the experimental bond angles are taken as input for calculating both the double-exchange hoppings and superexchange intensity (see Methods section and Supplementary Note 2 ). By using a set of proper parameters (see Methods section), the T -dependence of magnetization obtained in the simulation are shown in Fig. 4a . With decreasing T , the N =2 case shows a quenched magnetization, while others become FM finally. The N =4 and 6 cases give stronger FM (larger M and higher T c ) than the N =3 case. Despite the FM ground state, all of them are insulating. All these features agree with the experimental observations, implying that our model simulation captures the main physics. For comparison, the simulation is re-done for all superlattices by adopting the bond angles of the N =6 case. As shown in Fig. 4b , the simulated magnetizations display contrasting results: all of them are strongly FM with similar T c and saturated M s . The qualitative differences between Fig. 4a,b suggest the crucial role of bond angles, or OOR, to determine the magnetism of LaMnO 3 layers. 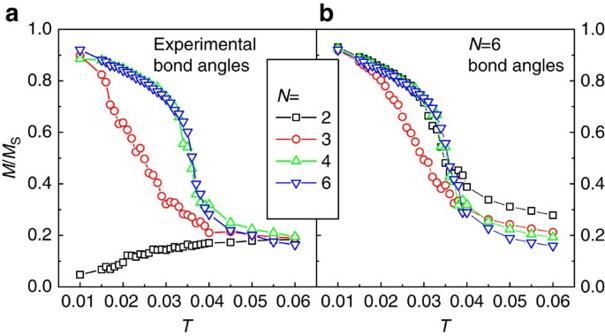Figure 4: Temperature-dependent magnetization per Mn obtained from Monte–Carlo simulation of the double-exchange model. (a) Calculated results using the experimental bond angles from each (LaMnO3)N/(SrTiO3)Nsuperlattice. (b) Calculated results using theN=6 bond angles for allN.MSis the saturated magnetization of 4μB. The non-zero residual magnetism at high temperature aboveTCis due to the finite size effect of simulated lattices. Figure 4: Temperature-dependent magnetization per Mn obtained from Monte–Carlo simulation of the double-exchange model. ( a ) Calculated results using the experimental bond angles from each (LaMnO 3 ) N /(SrTiO 3 ) N superlattice. ( b ) Calculated results using the N =6 bond angles for all N . M S is the saturated magnetization of 4 μ B . The non-zero residual magnetism at high temperature above T C is due to the finite size effect of simulated lattices. Full size image In addition, the pure dimensional effect is also further checked since in the small N cases the two-dimensional-like LaMnO 3 layers might be different from the thicker three-dimensional-like one. However, our simulation result ( Supplementary Note 3 and Supplementary Fig. 6 ) rules out the dimensional reduction as the main driving force to the quenched magnetism in the N =2 superlattice. As a conclusion of above simulations, the suppressed magnetism in small N superlattices, especially N =2, is closely related to the decreased double-exchange interaction due to the enhanced OOR. Coherence and inhomogeneity of the octahedral rotation When the SrTiO 3 spacer layer is very thin, the OOR of LaMnO 3+ δ could be correlated between neighbouring super cells via rotation or slight structural distortion in the SrTiO 3 spacer layer, leading to coherent interference of OOR. Experimentally, we do observe interference fringes near the half-order Bragg peaks for N =2–6 samples ( Fig. 5a ), while the superlattice peaks remain clearly resolved. The absence of such features in the N =16 superlattice could be because of sample quality or phase mixture. The observation of thickness fringes implies that OOR are somewhat correlated across the interface, while the presence of the superlattice peaks indicates that the OOR is modulated by the superlattice period. The long-range structural coherence and large out-of-plane rotation in the N =2 superlattice conspire to give rise to in-plane structural modulations with large wavelength, as evidenced by clear satellite peaks, ~0.02 reciprocal lattice units away from the half-order peak along both H and K directions ( Fig. 5b ). No obvious satellite peaks can be seen for superlattices of N =4 and above. Similar long-range structure modulation has been observed in an (SrMnO 3 ) 2 /(LaMnO 3 ) 1 superlattice [34] . Possible explanations of the satellite peaks include, for example, distortion of oxygen octahedra, although more work is needed to confirm the underlying mechanism. 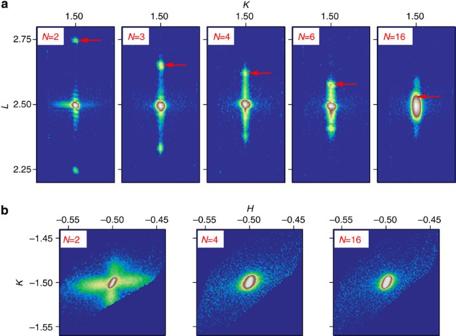Figure 5: Coherent interference and structural modulation from octahedral rotations in (LaMnO3+δ)N/(SrTiO3)Nsuperlattices. (a) LogarithmicKLintensity maps near (H,K,L)=(0.5,1.5,2.5) forN=2, 3, 4, 6, 16 superlattice samples. TheKrange in the map is ±0.05 in r.l.u. of SrTiO3. Red arrows indicate the expected positions for superlattice peaks. (b) Logarithmic in-planeHKintensity maps near (H,K,L)=(−0.5,−1.5,2.5) forN=2, 4, 16 superlattice samples. Figure 5: Coherent interference and structural modulation from octahedral rotations in (LaMnO 3+ δ ) N /(SrTiO 3 ) N superlattices. ( a ) Logarithmic KL intensity maps near ( H , K , L )=(0.5,1.5,2.5) for N =2, 3, 4, 6, 16 superlattice samples. The K range in the map is ±0.05 in r.l.u. of SrTiO 3 . Red arrows indicate the expected positions for superlattice peaks. ( b ) Logarithmic in-plane HK intensity maps near ( H , K , L )=(−0.5,−1.5,2.5) for N =2, 4, 16 superlattice samples. Full size image The fitting results in Fig. 3 describe the average effect of all the involved octahedra, including all MnO 6 and the interfacial TiO 6 . Although half-order peaks in N =2 sample should be dominated by interfacial OOR, inhomogeneity of OOR could exist for superlattices with larger N and affect the data analysis. On the other hand, as the X-ray scattering intensity from OOR scales roughly with the square of sine of the rotation angle (see equation (2) in Supplementary Note 1 ), we would expect that the observed half-order peaks mostly come from MnO 6 and the interfacial TiO 6 with large OOR. Therefore, even in the presence of OOR inhomogeneity, the fitting results obtained for N =2–6 superlattices should represent the systematic change of the rotation pattern in LaMnO 3+ δ layers: the derived bond angles in the N =2 superlattice feature the interfacial OOR; those in the N =4, 6 superlattices reflect an average bond angles of both the interfacial and inner LaMnO 3 layers. Note that the in-plane bond angles in Fig. 3 are larger than bulk LaMnO 3 , which could be possibly attributed to the strain or hole doping, or an averaging effect from interfacial TiO 6 octahedra with larger bond angles. In general, a rigorous model incorporating all the separate rotations at different layers is very difficult to verify from X-ray data. However, the simple OOR model with few fitting parameters describes the experimental data fairly well, implying that the model is a reliable approximation and captures the essential physics. Additional proof from (LaMnO 3+ δ ) N /(SrTiO 3 ) 2 superlattices To further test the validity of simple OOR model and confirm the correlation between OOR and FM, we performed similar measurements and analysis for another set of (LaMnO 3+ δ ) N /(SrTiO 3 ) 2 ( N =2, 4, 6) superlattices with constant SrTiO 3 thickness ( Fig. 6 and Supplementary Table 2 ). The constant and thin SrTiO 3 thickness in the supercell enables the observation of a more systematic evolution of the OOR pattern, and minimizes the inhomogeneity of OOR across the superlattice. Again only half-order peaks with all H , K , L being half-integers are observed, whose experimental intensity are summarized in Fig. 6a , together with the fits based on simple OOR model. The good fits again indicate that this simple model works fairly well. The deduced bond lengths and angles are summarized in Fig. 6b . The in-plane Mn–O–Mn bond angle shows an increase of ~5° from N =2–6, while the out-of-plane bond angle decreases ~3°. The M s for both sets of superlattices are plotted in Fig. 6c for comparison. It is interesting to see that M s in the (LaMnO 3+ δ ) N /(SrTiO 3 ) 2 superlattices show similar increase with N as (LaMnO 3+ δ ) N /(SrTiO 3 ) N superlattices, albeit in a smaller magnitude. This seems to correlate well with the change of the magnitude in the Mn–O–Mn bond angles (compare Figs 3c and 6b ). Therefore, these new results provide another direct experimental evidence of the correlation between OOR and FM in these superlattices. 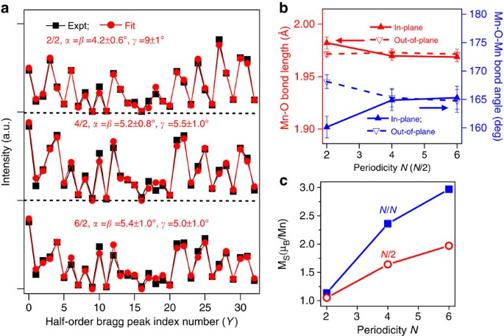Figure 6: The octahedral rotation and the saturation magnetization for (LaMnO3+δ)N/(SrTiO3)2(N/2) superlattices. (a) Experimental (Expt.) half-order Bragg peak intensities (black squares) compared with model fits (red dots) for (LaMnO3+δ)N/(SrTiO3)2superlattices (N/2). From top to bottom are results fromN=2 (2/2),N=4 (4/2) andN=6 (6/2) superlattices, respectively. The Half-order Bragg peaks are labelled by the index number (Y), with its correspondingH,K,Lvalues shown inSupplementary Table 2. Note that only half-order peaks with allH,K,Lbeing half-integer are observed and shown here. The best fit values ofαandγare shown with error bars. The data and fits are shifted vertically for display clarity. (b) In-plane (filled up triangles) and out-of-plane (hollow down triangles) Mn–O bond lengths (red) and Mn–O–Mn bond angles (blue) deduced from the octahedral rotation. The pseudocubic lattice constants are derived from the three-half-integer peaks similar toFig. 2f. (c) Comparison between the measured low temperature (T=5 K) saturation magnetizationMsof the (LaMnO3+δ)N/(SrTiO3)N(N/N) superlattices (blue squares) and the (LaMnO3+δ)N/(SrTiO3)2(N/2) superlattices (red hollow dots). Figure 6: The octahedral rotation and the saturation magnetization for (LaMnO 3+ δ ) N /(SrTiO 3 ) 2 ( N /2) superlattices. ( a ) Experimental (Expt.) half-order Bragg peak intensities (black squares) compared with model fits (red dots) for (LaMnO 3+ δ ) N /(SrTiO 3 ) 2 superlattices ( N /2). From top to bottom are results from N =2 (2/2), N =4 (4/2) and N =6 (6/2) superlattices, respectively. The Half-order Bragg peaks are labelled by the index number ( Y ), with its corresponding H , K , L values shown in Supplementary Table 2 . Note that only half-order peaks with all H , K , L being half-integer are observed and shown here. The best fit values of α and γ are shown with error bars. The data and fits are shifted vertically for display clarity. ( b ) In-plane (filled up triangles) and out-of-plane (hollow down triangles) Mn–O bond lengths (red) and Mn–O–Mn bond angles (blue) deduced from the octahedral rotation. The pseudocubic lattice constants are derived from the three-half-integer peaks similar to Fig. 2f . ( c ) Comparison between the measured low temperature ( T =5 K) saturation magnetization M s of the (LaMnO 3+ δ ) N /(SrTiO 3 ) N ( N / N ) superlattices (blue squares) and the (LaMnO 3+ δ ) N /(SrTiO 3 ) 2 ( N /2) superlattices (red hollow dots). Full size image The observed change of the Mn–O–Mn bond angles for small N superlattices could be understood in terms of the OOR proximity effect: the octahedral connectivity in the out-of-plane direction requires the bond angle of interfacial layers to be large in the vertical direction; this results in a reduction of in-plane bond angle (via an enhanced c axis rotation) as predicted by density-functional theory calculations [10] . In a structurally similar (4 unit cell (u.c.) LaNiO 3 /3 u.c. SrTiO 3 ) N superlattice (bulk LaNiO 3 has an a - a - a - rotation), enhanced bond angle along the c axis accompanied by reductions of bond angle along in-plane axes has been observed in the interfacial LaNiO 3 layer, which was explained by a combined effect of octahedral connectivity and epitaxial strain [35] . A careful examination of our data suggests that the two cases could be similar, as evidenced by a larger pseudocubic c lattice constant in both cases, that is, c p / a p >1 ( Fig. 2f ). In our case, the increase of the out-of-plane Mn–O–Mn bond angle with decreasing N is apparent in (LaMnO 3+ δ ) N /(SrTiO 3 ) 2 superlattices and less obvious in (LaMnO 3+ δ ) N /(SrTiO 3 ) N superlattices. The detailed quantitative difference has not yet been understood. The current finding may provide a new insight to the ‘dead’ layer issue that are commonly found at the interface between manganite oxides and many perovskite substrates [36] , and has attracted renewed interests. In recent studies, orbital ordering, [37] polar discontinuity [38] , [39] , magnetic coupling to the titanate layer, [40] stoichiometry [41] , [42] and so on, have all been evidenced to couple to the interface magnetic property of the manganite layer, while a unified scenario is still lacking. Some recent studies on La 0.67 Sr 0.33 MnO 3 /SrTiO 3 interfaces have merged on the finding of increased amount of Mn 3+ near the interface [43] , [44] , [45] and 3 z 2 − r 2 orbital ordering irrespective of the strained state [37] , [45] , [46] . Our study suggests that the reconstructed OOR at the interface is another nontrivial factor in determining the interfacial magnetic property. Sample growth and magnetic measurements The (LaMnO 3+ δ ) N /(SrTiO 3 ) N ( N =2, 3, 4, 6, 8, 16) superlattices, (LaMnO 3+ δ ) N /(SrTiO 3 ) 2 ( N =2, 4, 6) superlattices and thin-film LaMnO 3+ δ samples were grown on SrTiO 3 (001) single-crystalline substrates using stoichiometric LaMnO 3 and SrTiO 3 targets by RHEED-assisted pulsed laser deposition. Substrates with atomically flat TiO 2 termination were obtained after buffered Hydrofluoric (HF) acid etching and annealing at 950 °C for 1 h. All samples were grown at the substrate temperature of 700 °C with an oxygen pressure of 3 × 10 −5 mbar. The laser energy density was ~1 J cm −2 and the pulse frequency was 1 Hz. The superlattice periodic structure was controlled by monitoring RHEED oscillations and confirmed by the XRD measurements. After growth, samples were cooled down to room temperature subject to the same oxygen pressure as during growth. Magnetic measurements were performed in a Quantum Design VSM system from 4 to 200 K. The electric transport measurements are taken in a Quantum Design PPMS system and the results are shown in Supplementary Fig. 7 . XAFS measurements and analysis Mn K-edge X-ray absorption spectra were collected on the XAFS station (1W1B beamline) of the Beijing Synchrotron Radiation Facility. The X-ray energy was calibrated with a standard Mn foil. High harmonics were eliminated by detuning the double-crystal Si (111) monochromator. The XAFS measurements were conducted in fluorescence mode using a 19-element high-purity germanium solid-state detector at room temperature. In the XAFS study, we measured the Mn K -edge spectra of polycrystalline Mn 2 O 3 and MnO 2 powder samples as references to the superlattices and the LaMnO 3+ δ thin film. In ref. 47 , Mn K -edge spectra of stoichiometric MnO 2 , Mn 2 O 3 , LaMnO 3 and CaMnO 3 were measured in the same condition. By aligning the spectra of the Mn 2 O 3 and MnO 2 of our study to those in ref. 47 , we are able to correct the energy scale and make accurate comparison of the superlattice and LaMnO 3+ δ thin-film spectra to the stoichiometric LaMnO 3 and CaMnO 3 spectra from ref. 47 ( Supplementary Fig. 3 ), by shifting our measured spectra with the amount of energy difference discussed above. The threshold energy ( E 0 ) of the K-edge depends on the Mn valence and continuously increases with increasing Mn valence [48] . The dependence of E 0 on Mn valence can be roughly fitted by a linear law. E 0 is identified by finding the energy at which the first-order differentiation d I /d E is the maximum and the second-order differentiation d I 2 /d E 2 is zero. I is the intensity of the absorption spectra and E is the X-ray energy. In ref. 47 , E 0 of Mn 3+ in LaMnO 3 is 6,450.6 eV and E 0 of Mn 4+ in CaMnO 3 is 6,454.8 eV. E 0 of the superlattices and the LaMnO 3+ δ thin film is marked in the inset of Supplementary Fig. 3a . The Mn valence of the superlattice samples and the thin-film LaMnO 3+ δ sample is inferred using the linear relation between E 0 and the valence of Mn, as shown in Supplementary Fig. 3b . XRD measurements Synchrotron XRD measurements were carried out at Sector 33BM of the Advanced Photon Source at room temperature, using 15 keV X-rays ( λ =0.8266 Å). Geometric corrections and background subtraction are taken into account for all the data. All the reciprocal space maps, displayed as image plots using a logarithmic intensity scaling, were generated as k-space projections from the three-dimensional volume data sets acquired during a single linear scan using a Pilatus 100 K area detector, without background subtraction. Double-exchange model and Monte–Carlo simulation Our model includes the double-exchange between two e g orbitals, electron-lattice coupling (both the Jahn–Teller modes and breathing mode), and nearest neighbour superexchange between t 2g spins. In past decades, this model has been proved to be successful to give a realistic description of manganites [49] . Customarily, the double-exchange hopping coefficient t 0 (~0.4–0.5 eV) refs 49 , 50 is taken as the energy unit all through the simulation. According to previous literature, a set of parameter ( J AF 0 , λ ) is chosen as (0.095,1.2) in our simulation if not noted explicitly, where J AF 0 is the coefficient of superexchange for 180° Mn–O–Mn bond angle and λ is the coefficient for electron-lattice coupling. Then the effects of Mn–O–Mn bending bonds to both the double-exchange and superexchange have been taken into account, the formulas of which can be found in Supplementary Note 2 . The lattice used in Monte–Carlo simulation is 4 × 4 × N . For exchanges, the boundary conditions are periodic in the x – y plane but open along the z axis to simulate the isolated manganite layers, while for lattice distortions, full periodic boundary conditions are imposed since the oxygen octahedra are all complete in the superlattices. Owing to the strain effect, the LaMnO 3 thin film on SrTiO 3 gives quite close values (3.905/3.905/~3.91 Å) between pseudocubic lattice constants ( a / b / c ). For simplicity, a cubic structure is adopted in our simulation, which is a reasonable approximation. The valence of Mn is fixed as +3, without any non-stoichiometry or charge transfer between Mn and Ti. Thus, our model is a clean system to verify the effect of OOR. The model Hamiltonian is studied by a sophisticated method in combination of exact diagonazition of the Fermion sector and Monte–Carlo simulation of spins and lattice degrees of freedom. The magnetizations shown in Fig. 4 are extracted from the spin structure factor at the Γ point. Kubo conductances are also calculated, which shows insulating behaviour for all studied superlattices with above parameters. More details of our model used here can be found in Supplementary Note 2 and references therein. To solve the Hamiltonian described in Supplementary Note 2 , the Fermion sector, including the double-exchange and electron-lattice coupling, is solved by exact diagonazition. Although the spin and lattice degrees of freedom (S and Q) are simulated by Monte–Carlo method [49] , [51] . 1 × 10 4 Monte–Carlo steps are used for thermal equilibrium and the following 1 × 10 4 steps are used for measurement. The Kubo conductance is calculated based on the linear response theory [52] . The spin structure factor is calculated as: where V is the number of total sites, or namely the volume. Periodic boundary conditions are used here. The magnetization shown in Fig. 4 is calculated as . How to cite this article: Zhai, X. et al. Correlating interfacial octahedral rotations with magnetism in (LaMnO 3+ δ ) N /(SrTiO 3 ) N superlattices. Nat. Commun. 5:4283 doi: 10.1038/ncomms5283 (2014).